Desorption kinetics from a surface derived from direct imaging of the adsorbate layer There are numerous indications that adsorbed particles on a surface do not desorb statistically, but that their spatial distribution is important. Evidence almost exclusively comes from temperature-programmed desorption, the standard method for measuring desorption rates. However, this method, as a kinetics experiment, cannot uniquely prove an atomic mechanism. Here we report a low-energy electron microscopy investigation in which a surface is microscopically imaged while simultaneously temperature-programmed desorption is recorded. The data show that during desorption of oxygen molecules from a silver single crystal surface, islands of oxygen atoms are present. By correlating the microscopy and the kinetics data, a model is derived that includes the shapes of the islands and assumes that the oxygen molecules desorb from the island edges. The model quantitatively reproduces the complex desorption kinetics, confirming that desorption is affected by islands and that the often used mean-field treatment is inappropriate. When adsorbed particles desorb from a surface, for example, the molecules produced in a catalytic reaction, this is mostly regarded as a process of uniform, statistically independent events. The desorption rate is then proportional to the coverage Θ. For recombinative desorption of dissociatively adsorbed particles, the rate is proportional to Θ 2 if the events are uniform and statistically independent. This model, which is equivalent to a mean-field treatment of the desorption, goes back to Irving Langmuir [1] , but is still widely used for analysing kinetic data in modern surface kinetics, for example, in microkinetic models of heterogeneous catalysis [2] , [3] . On the other hand, there are numerous indications that the mean-field treatment of desorption is not generally valid. Temperature-programmed desorption (TPD), the standard method for determining desorption kinetics, hardly ever shows pure Langmuir behaviour. The desorption order, the exponent m in the desorption rate law, , is often a fractional number rather than the expected m =1 or 2, and the desorption peaks in TPD can have unexpected widths or symmetries or be split into multiple peaks. Reasons for non-Langmuir behaviour during desorption have been discussed since the 1970s [4] , [5] and were studied more recently by statistical mechanical treatments [6] and by kinetic Monte-Carlo simulations [7] , [8] , [9] . It has been shown that multiple adsorption states and interactions between the particles affect the kinetics [6] , [8] , [9] . Particularly strong deviations may occur if adsorbed particles form two-dimensional (2D) islands, as is the case for most adsorbates at some temperature. Depending on the mobility of the adsorbate layer, which determines whether it is in 2D equilibrium during desorption or not, the consequences will be different [7] . If the mobility is restricted, one expects that only the particles at the perimeters of islands desorb, which should lead to m =1/2. However, fractional desorption orders can also be explained by coverage-dependent lateral interactions in uniform adlayers. Conversely, islands need not lead to m =1/2 if the islands are in equilibrium with a dilute 2D phase, and observations of zero-order desorption have been explained in this way [10] , [11] , [12] . The difficulties of imaging an adsorbate layer during desorption have so far almost completely prevented experimental access to these effects. Usually, the TPD traces are the only data available, and because there are so many unknown complexities on the microscopic level, the true underlying desorption mechanism cannot be derived in a unique way. One faces the same logical asymmetry problem as with any kinetics experiment: if the microscopic mechanism of a chemical process is known, it can be uniquely translated into the kinetics, whereas the reverse is not possible, kinetics cannot uniquely be translated into a microscopic mechanism. In an experiment that overcomes this problem, we have used low-energy electron microscopy (LEEM) to directly view the surface morphology during desorption. The system studied, adsorbed oxygen atoms on an Ag(111) surface, is known for its strong desorption anomalies in TPD, namely, the O 2 desorption peak does not show the shift to lower temperature with initial O coverage expected for recombinative desorption, and it can split into two peaks [13] , [14] , [15] . The binding of oxygen to silver surfaces plays an important role in the Ag-catalysed synthesis of ethylene oxide [16] , [17] . We show that the anomalies in the oxygen desorption are explained by the fragmentation of the O adlayer into islands during O 2 desorption. Using the observed complex island morphology, we derive a model that quantitatively describes the desorption kinetics. LEEM and photoemission electron microscopy (PEEM) have been used before to investigate 2D phase transitions on surfaces [18] , [19] and also to study desorption and sublimation from surfaces [18] , [20] , [21] , [22] , [23] . However, there are no studies that quantitatively correlate microscopic processes with desorption kinetics measured by TPD. In addition, the observed heterogeneity of the Ag(111) surface, which affects the desorption kinetics of adsorbed oxygen, is also highly relevant for catalytic reactions. For the Ag-catalysed conversion of ethylene to give ethylene oxide, it has been shown that a heterogeneous surface containing different oxygen species is of major importance [16] , [17] , [24] . Combination of LEEM and TPD The experiments were performed with the spectroscopic photoemission and LEEM instrument at Elettra in Trieste [25] . Oxygen was adsorbed on Ag(111) by dosing NO 2 at T ≥450 K. NO 2 decomposes into oxygen atoms and NO, and the NO desorbs. This method avoids the large gas exposures required when O 2 is used [14] . The adsorbed O atoms form an ordered surface structure with a (4 × 4) lattice. It involves a reconstruction of the Ag(111) surface in which the structure of the topmost metal layer is modified, creating more favourable sites for the O atoms [26] , [27] , [28] . For the TPD experiments, the sample temperature was linearly ramped up ( T = T 0 + βt , with initial temperature T 0 and heating rate β ), and the desorbing O 2 was monitored with a quadrupole mass spectrometer (QMS). TPD experiments The five TPD traces shown in Fig. 1a–e were recorded in consecutive experiments. After each TPD, the same amount of oxygen was adsorbed at 490 K, and a further TPD trace was recorded, without intermediate sample preparation. At first, O 2 desorbs in one peak at ~520 K, then a second peak splits off and shifts to higher temperatures. Fits to the TPD traces with second-order desorption, expected for recombinative desorption of O 2 , fail completely for any parameter set, even when only one peak is present (green curve in Fig. 1a ). A fit with first-order desorption, using a fixed preexponential factor of 1 × 10 13 s −1 , gave a desorption energy of 1.51 eV, but very bad agreement. Only slightly better agreement was achieved when the desorption energy was kept fixed at 1.66 eV, the value obtained from our analysis below, which gave a preexponential factor of 1.4 × 10 14 s −1 (red curve in Fig. 1a ). A good first-order fit was only obtained with apparently unreasonable parameters, for example, with a desorption energy of 2.38 eV and a preexponential factor of 3.6 × 10 21 s −1 . 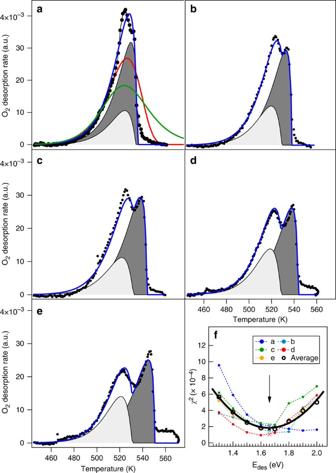Figure 1: TPDs of oxygen from Ag(111). (a–e) TPD traces, showing them/z=32 signal from the QMS (black dots), measured in a series of consecutive experiments (heating rates 0.50, 0.50, 0.48, 0.40 and 0.42 K s−1). Fits to the island perimeter model (blue), with contributions by the smaller islands (light grey shading) and larger islands (dark grey shading). Red line ina: fit withm=1,εdes=1.66 eV andν=1.4 × 1014s−1. Green line: fit withm=2,εdes=1.66 eV andν=3.1 × 1014s−1. (f) Goodness of fit for a series ofν/εdescombinations for the individual TPDs and average. Figure 1: TPDs of oxygen from Ag(111). ( a – e ) TPD traces, showing the m / z =32 signal from the QMS (black dots), measured in a series of consecutive experiments (heating rates 0.50, 0.50, 0.48, 0.40 and 0.42 K s −1 ). Fits to the island perimeter model (blue), with contributions by the smaller islands (light grey shading) and larger islands (dark grey shading). Red line in a : fit with m =1, ε des =1.66 eV and ν =1.4 × 10 14 s −1 . Green line: fit with m =2, ε des =1.66 eV and ν =3.1 × 10 14 s −1 . ( f ) Goodness of fit for a series of ν / ε des combinations for the individual TPDs and average. Full size image LEEM experiments during isothermal desorption We find that the complexity of the TPD data is reflected by the microstructure in LEEM. 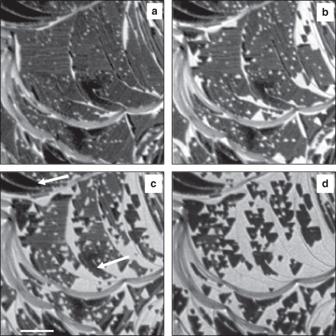Figure 2: LEEM images during isothermal desorption of oxygen. The images were recorded at 487 K as the NO2pressure was lowered and oxygen desorbed isothermally. Approximately 190 s between images. Black: well-ordered (4 × 4)O structure, dark grey: (4 × 4)O structure with linear defects, light grey: Ag(1 × 1) surface. Arrows indicate two of the large islands of the well-ordered (4 × 4)O structure (black) during decay. FOV, 4.8 μm; scale bar, 1 μm; and bright field imaging at 19 eV (Supplementary movie 1). Figure 2 shows an isothermal desorption experiment in which steady-state conditions were initially adjusted at T =487 K by tuning the NO 2 pressure such that adsorption and O 2 desorp-tion rates were balanced. Then, the NO 2 pressure was lowered, so that the oxygen coverage decreased, but more slowly than in TPD, so that the data showed the structure changes with higher resolution. Figure 2: LEEM images during isothermal desorption of oxygen. The images were recorded at 487 K as the NO 2 pressure was lowered and oxygen desorbed isothermally. Approximately 190 s between images. Black: well-ordered (4 × 4)O structure, dark grey: (4 × 4)O structure with linear defects, light grey: Ag(1 × 1) surface. Arrows indicate two of the large islands of the well-ordered (4 × 4)O structure (black) during decay. FOV, 4.8 μm; scale bar, 1 μm; and bright field imaging at 19 eV ( Supplementary movie 1 ). Full size image The dark areas are oxygen covered and the bright regions are clean Ag(111). In the beginning, the dark regions show two different brightness levels, one almost black and the other dark grey with faint streaks ( Fig. 2a ). Both areas show a (4 × 4) diffraction pattern. The black areas correspond to a perfect (4 × 4)O structure. The dark grey, streaky areas are explained by a (4 × 4)O structure with oxygen vacancies. Using scanning tunnelling microscopy it has been shown that partial removal of oxygen from the (4 × 4)O phase leads to characteristic linear domain boundaries [29] . These can account for the streaks resolved by LEEM. During oxygen desorption, the streaks disappear, indicating that the defect-rich (4 × 4)O structure orders, and at the same time these areas decompose into many small, triangular (4 × 4)O islands, whereas the initially well-ordered (4 × 4)O structure still forms large, coherent islands (arrows in Fig. 2c ). 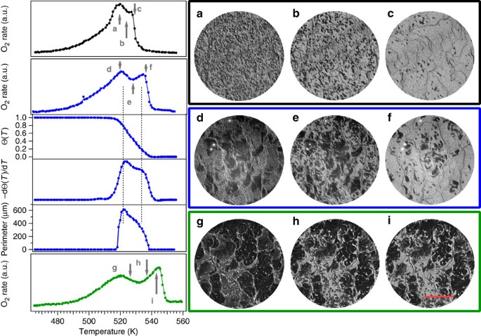Figure 3: LEEM images during TPD of oxygen. Three O2TPDs (black, blue and green data) and still images from simultaneously recorded LEEM movies (1 frame per 2 s, heating rates 0.50, 0.48 and 0.42 K s−1); corresponding time instants are marked. The (4 × 4)O islands appear dark. FOV, 15 μm; scale bar, 5 μm (in image i); and bright field imaging at 19 eV. Also shown is an analysis of the second LEEM series (blue data): O coverage Θ(T), derivative −dΘ(T)/dTand total perimeter of all islands (Supplementary movies 2 and 3). LEEM experiments during TPD Figure 3 shows three consecutive TPD experiments (frames on the left) with simultaneously recorded LEEM data (frames on the right). From each of the three LEEM movies, three frames are shown, with letters (a, b, c and so on) marking the same time instants in the TPD traces. The LEEM data were noisier than in the constant temperature experiment ( Fig. 2 ) because of the shorter acquisition times. Nevertheless, one can still recognize the smaller and larger islands. In the first experiment (top row), the LEEM frames almost exclusively show one island type (the—relatively—larger islands; the smaller islands are at the resolution limit), and the simultaneous TPD trace (top frame, black data points) shows one peak at time instant a and a shoulder at c. In the second experiment (centre row), both smaller and larger islands are visible, and in the TPD trace (second frame, blue data points) a second peak splits off (at f). In the third experiment (bottom row) the larger islands are further enlarged, and the second TPD peak (green data points) has shifted to a higher temperature (at i). The two peaks in the TPDs are obviously correlated with the smaller and larger islands. They are not caused by different phases—both island types have the (4 × 4)O structure—but by their different morphologies. Both types of islands become larger from run to run, which is caused by a decreasing number of defects in the originally formed (4 × 4)O structure. Figure 3: LEEM images during TPD of oxygen. Three O 2 TPDs (black, blue and green data) and still images from simultaneously recorded LEEM movies (1 frame per 2 s, heating rates 0.50, 0.48 and 0.42 K s −1 ); corresponding time instants are marked. The (4 × 4)O islands appear dark. FOV, 15 μm; scale bar, 5 μm (in image i); and bright field imaging at 19 eV. Also shown is an analysis of the second LEEM series (blue data): O coverage Θ( T ), derivative −dΘ( T )/d T and total perimeter of all islands ( Supplementary movies 2 and 3 ). Full size image That there are two (4 × 4) areas with different vacancy concentrations is explained by small amounts of oxygen in the subsurface region from which vacancies in the (4 × 4) phase can be filled during preparation. During the repeated TPDs, the subsurface oxygen accumulates but remains below the spectroscopically detectable limits. The additional oxygen is indicated by the slightly increasing base line on the high-temperature side of the desorption peaks ( Fig. 1 ). The maximum amount, reached in the last experiment ( Fig. 1e ), is about 6% of the totally desorbed oxygen, so that it affects the desorption kinetics only indirectly via the defect density in the (4 × 4) layer. An alternative explanation could be an impurity at the Ag(111) surface, which binds oxygen more strongly by somehow modifying the electronic structure of the surface, given this impurity remains below spectroscopic detection limits. However, we found a way to greatly accumulate the postulated oxygen subsurface species, so that it became spectroscopically detectable [30] , whereas other impurities were still absent. Hence, although we initially considered foreign elements and intensively searched for such a possibility [31] , we now consider it as highly unlikely. Analysis of the LEEM data To explore whether the evolution of the islands correlates with the TPD peaks in a quantitative way, the (4 × 4)O area, A 4 × 4 , was determined from the LEEM data. Divided by the field-of-view (FOV) area, A FOV , of the imaged surface, A 4 × 4 is a measure of the oxygen coverage, Θ. The thus determined Θ( T ) curve is shown in Fig. 3 for the second experiment (blue data points). The negative derivative, , should be proportional to the desorption rate, the quantity measured by TPD. This is indeed the case, ( Fig. 3 , blue data points) shows a double peak at the same temperatures as the peaks in the TPD trace of the same experiment ( Fig. 3 ). (The time derivative was replaced by the equivalent temperature derivative.) That the slowly increasing desorption rate at the low-temperature side of the TPD peak does not appear in the plot results from the fact that at the beginning of the temperature ramp the LEEM instrument does not spatially resolve the islands. Only the overall intensity of the LEEM data changed, and separate islands were resolved only shortly before the peak. Also the total perimeter length was determined from the LEEM data ( Fig. 3 , lowest of the blue data point frames). The analysis was performed by attributing grey levels to the islands and the uncovered areas and measuring the length of the boundary between the two areas. Because of the uncertain exact position of the threshold between the two levels, the absolute perimeter length and the detailed curve shape were correlated with relatively large errors. However, independently of the parameters of the analysis, the resulting curve showed a double-peaked structure with a maximum and a shoulder at exactly the same temperatures as the maxima in the TPD. Rate equation These observations were used to formulate a rate law to derive the TPD spectra. The desorption rate of oxygen from the total (4 × 4)O area on the FOV is given by the (negative) decay rate of an average single island of the smaller type (a) times the number N a of these islands in the field of view, plus the corresponding term for the islands of the larger type (b): A a and A b are the areas of an average single a or b island. For the decay rate ( i =a or b) of an individual a or b island, a Polanyi–Wigner ansatz was made: The (negative) decay rate of an individual island is given by an Arrhenius term (frequency factor ν , desorption energy ε des , temperature T , Boltzmann constant k ) times an area-dependent term (desorption order m i ). β is the heating rate, C i a factor containing geometric parameters. Equation (2) was numerically integrated, the computed rates and were substituted into equation (1) and the resulting rate versus temperature curve was fitted to the experimental TPD data. Almost perfect agreement was obtained ( Fig. 1 ). Of the parameters used for the fits, N a and N b were extracted from the LEEM data, C a and C b were geometric parameters (see Methods, equations (6) and (7)) and β was given by the experiment. m a , the desorption order of the smaller islands, was kept fixed at 1/2. Half-order desorption is expected if oxygen desorbs from island perimeters. The perimeter length is proportional to the square root of the area given the islands are compact and shrink uniformly, which is the case for the smaller islands. The alternative desorption from a rapid pre-equilibrium between the islands and O atoms on the unreconstructed surface [10] , [11] , [12] , which can lead to m =0, can be ruled out from the observed correlation of island perimeters and desorption rates. The larger islands were more difficult to treat analytically because of their irregular shapes and because they develop lobes during their decay (see, for example, the third experiment in Fig. 3 ). As a result, the perimeter of a large island decreases less rapidly than for m =1/2, and initially it may even increase if the lobes develop faster than the area shrinks. We mimicked this behaviour by using an exponent m b <1/2, and for the whole TPD data set, m b =0.3 proved to be a good value that was therefore held constant for all fits. For the two other unknown parameters, ν and ε des , several combinations led to good fits of individual experiments ( Fig. 1f ). However, when all TPD experiments were combined, a clear goodness-of-fit minimum was obtained for ν =5 × 10 16 s −1 and ε des =1.66±0.08 eV, for both peaks. The high preexponential factor may be explained by a mobile transition state of the O 2 molecules desorbing from the island perimeters that have a higher partition function. For ε des , previous TPD investigations of Ag(111)/O gave values between 1.35 and 2.68 eV, but the analyses were based on an assumed first or second-order desorption, which is not confirmed here [13] , [15] , [32] , [33] . (2.68 eV was considered unphysical by the authors [15] .) Density functional theory calculations gave a binding energy of atomic oxygen in the (4 × 4)O structure of 3.5 eV [34] , in good agreement with the value of 3.4 eV that corresponds to the (molecular) desorption energy of 1.66 eV ( ε ad (O)=1/2 × [ ε des (O 2 )+ ε diss (O 2 )]=1/2 × [1.66+ 5.15 eV]=3.4 eV). Alternatively, the O 2 molecules may desorb from a diffusion ‘seam’ of O atoms around the (4 × 4)O islands. Diffusion followed by desorption has been resolved by PEEM during sublimation of Ag from a Si(001) surface [22] . (Otherwise this system is quite different, as desorption occurs from a second 2D solid phase around the Ag islands.) We have made an effort to resolve such an enhanced concentration of O atoms around the (4 × 4)O islands by mirror electron microscopy (MEM) and area-selected (μ-probe) X-ray photoelectron spectroscopy (XPS), using the same instrument as for LEEM. However, within the sensitivity and spatial resolution limits of these techniques (in this particular experiment, the MEM sensitivity for adsorbed O atoms was better than 0.03 monolayers, the resolution considerably better than 1 μm, the limits in the μ-probe XPS were similar), no such seam was resolved. If one estimates the diffusion length of adsorbed O atoms (using 10–20% of the adsorption energy for the diffusion barrier [35] , the desorption maximum at 520 K and the TPD time scale of 10 s), one obtains values between 1.5 and 65 μm, so that such a seam could have been resolved. As this was not the case, such a mechanism appears less likely here. Of course, for the observed scaling of the desorption rate with the island perimeter, it does not make a difference whether the O atoms directly recombine at the island edges or first detach from the edges and then recombine in a narrow diffusion seam of O atoms around the islands. Steady-state experiments To verify the model of perimeter-limited desorption kinetics, ν and ε des were also determined in an independent experiment ( Fig. 4 ). The sample was dosed with NO 2 at constant pressures and temperatures between 450 and 540 K. At each temperature, the pressure was adjusted such that the LEEM showed an unchanging partial coverage of (4 × 4)O islands, corresponding to steady-state adsorption/desorption conditions. 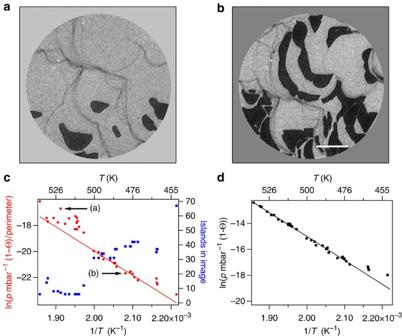Figure 4: LEEM during steady-state oxygen adsorption and desorption. LEEM images (a) at 523 K and 1.7 × 10−6mbar of NO2, and (b) at 481 K and 8.3 × 10−8mbar of NO2(FOV, 10 μm; scale bar, 2 μm; and bright field imaging at 19 eV). (c) Logarithm ofp(NO2), normalized by the uncovered surface area andltotal, versus 1/T(red), and island numbers in the imaged area versus 1/T(blue). (d) Logarithm ofp(NO2), normalized by the uncovered surface area, versus 1/T. The last four data points at low temperatures were not included because of clean-off reactions. The oxygen adsorption rate by NO 2 decomposition (gas temperature T gas =300 K) Figure 4: LEEM during steady-state oxygen adsorption and desorption. LEEM images ( a ) at 523 K and 1.7 × 10 −6 mbar of NO 2 , and ( b ) at 481 K and 8.3 × 10 −8 mbar of NO 2 (FOV, 10 μm; scale bar, 2 μm; and bright field imaging at 19 eV). ( c ) Logarithm of p (NO 2 ), normalized by the uncovered surface area and l total , versus 1/ T (red), and island numbers in the imaged area versus 1/ T (blue). ( d ) Logarithm of p (NO 2 ), normalized by the uncovered surface area, versus 1/ T . The last four data points at low temperatures were not included because of clean-off reactions. Full size image was then exactly balanced by the O 2 desorption rate from the perimeters of the (4 × 4)O islands: n ad is the area concentration of O atoms, p (NO 2 ) the pressure, m (NO 2 ) the molecular mass of NO 2 , s 0 the reactive sticking coefficient on the empty Ag surface and the fraction of empty surface. C in equation (4) contains geometric parameters, and l total is the total island perimeter length determined in the field of view of the LEEM (see Methods). (We do not use equations (1) and (2) here because one cannot formulate an analytic expression in terms of island numbers for the few large and irregular islands under these conditions, while their perimeter length can be directly extracted from the LEEM data.) If the rates in equations (3) and (4) are identical, a plot of versus 1/ T should give a straight line. This is actually the case for temperatures lower than 500 K ( Fig. 4c ). ε des from the slope is 1.61±0.08 eV, ν =1.1 × 10 17±0.87 s −1 , in very good agreement with the TPD result. That the data at higher temperatures deviate from the straight line can be explained by the small numbers of islands under these conditions ( Fig. 4c , blue dots)). Then, relatively more oxygen desorbs from step bunches (these also contain oxygen), so that l total from the islands comes out too small. This can be compensated by assuming a constant l total in the series. Then, all data points fall on a straight line ( Fig. 4d ), with identical slope as in Fig. 4c ( ε des =1.61±0.04 eV), again in agreement with the TPD results. For the overall error, we estimate ±0.08 eV that includes an additional, systematic error from uncertainties in the temperature reading. All data can thus be consistently explained by desorption of oxygen from the edges of the islands. The reason is probably the reduced coordination of the O atoms at the edges, combined with the high recombination probability of the O atoms (which are on neighbouring sites in the (4 × 4)O structure). There had been many previous indications that the desorption kinetics of adsorbed particles is affected by island formation and that the simplistic mean-field treatment is incorrect. Because most particles attractively interact with each other, effects of islands had been quite plausible. However, the TPD data, usually the only data available, cannot strictly prove that a heterogeneous distribution of the particles plays a role because the information provided by macroscopic kinetics is insufficient. Here we have presented direct evidence for a massive role of islands in the desorption kinetics by microscopically visualizing the surface morphology during the desorption process. Because for most adsorbates island formation is known, we expect that this result is also valid for other systems. Experimental details The spectroscopic photoemission and LEEM instrument can perform X-ray PEEM, LEEM, MEM, μ-probe low-energy electron diffraction and μ-probe XPS. Acquisition rates were typically around 1 frame per s. The low rates were a consequence of the low electron fluxes chosen to prevent beam damage of the oxygen layer and the resulting low signal-to-noise ratio. The Ag(111) sample was cleaned by repeated Ar + sputtering and annealing to 773 K for 30 min until a sharp (1 × 1) low-energy electron diffraction pattern was observed and the surface was free of any contaminant as measured by μ-probe XPS. NO 2 (99.0 vol %) was dosed following a known recipe [14] . A capillary was placed with its opening close to the sample surface to minimize the amount of gas in the vacuum system. The quadrupole mass spectrometer was mounted at 74° from the sample surface normal but at a large distance such that basically the homogeneous gas pressure within the μ-metal-shielded compartment of the sample in front of the objective lens was recorded. Fits of the TPD data Equation (1) was used to calculate the oxygen desorption rate . A 4 × 4 is the total (4 × 4)O-covered area in the FOV area A FOV of the LEEM experiment (in the experiment shown in Fig. 3 , A FOV =176.7 μm 2 and diameter of FOV=15 μm). The island numbers N a and N b of the smaller (a) and larger islands (b) in the A FOV area, which were taken as constants in the individual TPDs, were evaluated by and . and are the areas of average single islands at the beginning of the experiments that were evaluated from the initial island diameters in the LEEM data. x a are the surface fractions initially covered by the defect-rich (4 × 4)O structure and (1− x a ) are the surface fractions initially covered by the well-ordered (4 × 4)O structure. The x a values were determined from the grey versus black (4 × 4)O areas at the beginning of the individual TPDs and from the areas covered by the smaller and larger islands after the desorption had started. The values of x a , the ratios and , and the resulting island numbers N a and N b for the individual experiments can be found in Supplementary Table 1 . Equation (2) was used to calculate the decay rates of the individual islands, , where i =a or b and A a and A b are the areas of average single a or b islands. The geometry parameters C i in equation (2) were obtained by formulating the decay rate of a single (4 × 4)O island of area A i that looses O atoms by O 2 desorption from its perimeter: k des is the desorption rate constant, the factor 2 accounts for the desorption of two O atoms per O 2 molecule, N ox is the number of O atoms at the island perimeter, A ox is the area of an average adsorption site of an O atom. N ox is given by the island perimeter length l i times the 1D density of the O atoms along the perimeter. The 1D density of the O atoms is 3/8 of the 1D density of the Ag atoms (which equals 1/ d , with d =2.89 Å, the lattice constant of the Ag(111) surface) because the oxygen coverage in the (4 × 4)O structure is Θ ox =3/8. Hence, . The average adsorption site area A ox of an O atom in the (4 × 4)O structure is . The perimeter length l i in the expression for N ox depends on the shape of the islands. The smaller islands ( i =a) are mainly equilateral triangles for which the perimeter length l a is related to the island area A a by . By substituting l a into N ox , and N ox and A ox into equation (5), dividing equation (5) by A FOV , replacing the time derivative by the temperature derivative and writing an Arrhenius equation for k des , one obtains equation (2) for i =a, and for the geometry constant: For the larger islands ( i =b), the island perimeter l b varies more slowly than by a square root function (as discussed above): , with m b <1/2. To obtain correct dimensions, one can write this as , so that A b is measured in μm 2 . Z is a dimensionless constant that accounts for the island shape. (For the above case of the triangular islands and m =1/2, Z would be 4.6.) By substituting the expression for l b in N ox and converting equation (5) in the same way as for the a islands, one obtains equation (2) for i =b, and for the geometry constant: A list of all parameters used in the fits can be found in Supplementary Table 2 . The β -values were kept at the fixed values given by the experiment. The x a values were determined within the restrictions given by the LEEM data in Supplementary Table 1 and were then kept fixed in the fits. and in Supplementary Tables 1 and 2 were extracted from the LEEM data and kept fixed, and m a was kept fixed at 0.5. A fixed value of m b =0.3 was found to fit the entire data set. Z was a free fit parameter, and values between 7 and 14 were found. Several combinations of the free fit parameters ν and ε des led to good fits of individual TPD experiments, but when the five experiments were combined, a clear goodness-of-fit minimum was obtained (see Fig. 1f ). The optimized values for the tuple ν =5 × 10 16 s −1 and ε des ~1.66 eV are listed in Supplementary Table 2 . Analysis of the steady-state experiments The parameters used in equation (3) were the following. The reactive sticking coefficient s 0 of NO 2 on Ag(111) is known to be high [14] , and we assumed a value of unity. p (NO 2 ) was the ion gauge reading, corrected by a factor 1/20, because the mass spectrometer indicated considerable decomposition of NO 2 at the chamber walls, so that a part of the total pressure was caused by NO. A 4 × 4 / A FOV was taken from the LEEM images. In equation (4), the geometry constant C relates the desorption rate to the length of the island perimeters in the FOV of the LEEM. It is given by . The factor of 2 accounts for the desorption of two O atoms per O 2 molecule, (3/8) times (1/d) is the 1D density of the O atoms along the edges of the (4 × 4)O islands and A FOV is the FOV area of the LEEM image (here 78.5 μm 2 for a FOV diameter of 10 μm). The analysis of the steady-state experiments is based on the assumption that the decomposition rate of NO 2 on the Ag surface (equation (3)) is balanced by the desorption rate of O 2 from the island perimeters (equation (4)). We have considered the alternative possibility that a pre-equilibrium is established between O atoms in the (4 × 4)O islands and a 2D lattice gas of O atoms on the (1 × 1)Ag surface, and that the O 2 molecules desorb from the 2D lattice gas. The energy for this process would be the sum of the (molecular) desorption energy from the lattice gas plus two times the energy difference between O in the lattice gas and the (4 × 4)O structure. This total energy is identical to the direct desorption energy from the (4 × 4)O structure, so that the steady-state experiment cannot discriminate between these two possibilities. How to cite this article: Günther, S. et al. Desorption kinetics from a surface derived from direct imaging of the adsorbate layer. Nat. Commun. 5:3853 doi: 10.1038/ncomms4853 (2014).